Hydrogen evolution from a copper(I) oxide photocathode coated with an amorphous molybdenum sulphide catalyst Concerns over climate change resulting from accumulation of anthropogenic carbon dioxide in the atmosphere and the uncertainty in the amount of recoverable fossil fuel reserves are driving forces for the development of renewable, carbon-neutral energy technologies. A promising clean solution is photoelectrochemical water splitting to produce hydrogen using abundant solar energy. Here we present a simple and scalable technique for the deposition of amorphous molybdenum sulphide films as hydrogen evolution catalyst onto protected copper(I) oxide films. The efficient extraction of excited electrons by the conformal catalyst film leads to photocurrents of up to −5.7 mA cm −2 at 0 V versus the reversible hydrogen electrode (pH 1.0) under simulated AM 1.5 solar illumination. Furthermore, the photocathode exhibits enhanced stability under acidic environments, whereas photocathodes with platinum nanoparticles as catalyst deactivate more rapidly under identical conditions. The work demonstrates the potential of earth-abundant light-harvesting material and catalysts for solar hydrogen production. Among the different sources of renewable energy (solar, wind, geothermal, biomass, hydroelectric, tidal and nuclear), only solar energy can be exploited on a scale commensurate with our growing energy requirements [1] . To be of practical interest, light harvesting must be coupled to efficient energy storage mechanisms to keep a constant energy supply during the periods of lower sunlight irradiation or at night. The storage of solar energy in the form of hydrogen is an ideal solution since hydrogen can be produced directly from water and converted back to electricity when needed using a fuel cell [2] . However, to collect solar energy on the terawatt scale, these devices need to be made of abundant materials and should ideally reach or exceed 10% solar-to-hydrogen (STH) conversion efficiencies. Photoelectrochemical (PEC) water splitting is attractive as it integrates in the same device both solar energy collection and water electrolysis. Like electrolysers, a PEC water-splitting device requires a catalyst for the hydrogen evolution reaction (HER). Ideal HER catalysts for PEC water splitting need not only produce hydrogen at low overpotentials but should also be optically transparent and form a stable electrical contact with the photoabsorbing material [3] , [4] . Pt, the best HER catalyst, is often deposited on a photocathode to promote PEC hydrogen production [5] , [6] , [7] , [8] , [9] , [10] . Pt is however too scarce and costly for a large-scale application. Thus, there is a growing interest to apply earth-abundant and non-precious metal HER catalysts for PEC hydrogen production [11] , [12] , [13] , [14] , [15] , [16] , [17] . We have developed amorphous molybdenum sulphide films as HER catalysts under acidic and neutral conditions [18] , [19] , [20] . While the as-prepared precatalysts might have various compositions depending on the synthetic procedure, the active species is the same and is best labelled as MoS 2+ x (ref. 20 ). The latter species has a Mo:S ratio close to 1:2, and contain both S 2 2− and S 2− ligands, with a S 2 2− :S 2− ratio of about 3:7 according to X-ray photoelectron spectroscopy (XPS) [20] . In this work, we derive a PEC method to deposit amorphous MoS 2+ x films onto surface-protected cuprous oxide photocathodes. Surface-protected Cu 2 O is arguably the state-of-the-art p -type oxide for PEC hydrogen production [10] and one of the most promising low-cost materials reported until now [21] . The direct band gap of Cu 2 O is suitable for capturing a large portion of the visible spectrum with a maximum STH efficiency of 18.1% based on the air mass (AM) 1.5 irradiance spectrum and a corresponding photocurrent of −14.7 mA cm −2 ( E g of Cu 2 O=2.0 eV) [10] . The MoS 2+ x catalyst shows activity comparable to that of previously reported Pt nanoparticles [10] , [22] and RuO x (ref. 23 ) deposited on the same surface-protected Cu 2 O photocathode. Moreover, compared with Pt, the MoS 2+ x catalyst gives an improved stability in PEC hydrogen production under acidic conditions. MoS 2+ x -coated Cu 2 O photocathode The Cu 2 O photocathode was prepared by an electrodeposition method similar to a previously reported protocol [22] , [24] . Detailed description of the experimental method is given in the Methods section. In brief, thin Cu 2 O films were deposited electrochemically from a lactate-stabilized copper sulphate-plating bath kept at 30 °C in a two-electrode configuration cell at a constant galvanostatic current density of −0.1 mA cm −2 for 105 min. In this work, a freshly polished titanium plate was used instead of a Pt mesh as counter electrode during the device preparation process to avoid Pt contamination. Subsequently, ultrathin protective layers of aluminium-doped zinc oxide (AZO, 20 nm) and titanium dioxide (TiO 2 ; 100 nm) were deposited by atomic layer deposition (ALD). The TiO 2 overlayer protects the buried Cu 2 O/AZO photovoltaic junction from the aqueous environment and transports the photogenerated electrons to the electrolyte where water reduction takes place [8] , [22] . 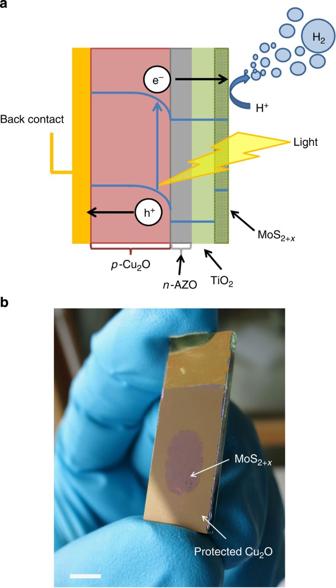Figure 1: MoS2+x-Cu2O photocathode. (a) Schematic structure of the surface-protected photocathode showing photon absorption and generation of an electron-hole pair in thep-Cu2O. The extraction of the excited electron through the TiO2-protective layer to produce hydrogen on the MoS2+xcatalyst is also illustrated. (b) A digital image of a MoS2+x-CA-Cu2O photocathode. Scale bar, 5 mm. The area covered with the MoS2+xcatalyst (66 μg cm−2) is in the middle of the photoelectrode and corresponds here to 0.48 cm2. Figure 1a is a schematic representation of photolytic HER from this device. Figure 1: MoS 2+ x -Cu 2 O photocathode. ( a ) Schematic structure of the surface-protected photocathode showing photon absorption and generation of an electron-hole pair in the p -Cu 2 O. The extraction of the excited electron through the TiO 2 -protective layer to produce hydrogen on the MoS 2+ x catalyst is also illustrated. ( b ) A digital image of a MoS 2+ x -CA-Cu 2 O photocathode. Scale bar, 5 mm. The area covered with the MoS 2+ x catalyst (66 μg cm −2 ) is in the middle of the photoelectrode and corresponds here to 0.48 cm 2 . Full size image The PEC deposition of MoS 2+ x was carried out utilizing unfiltered irradiation from a Xe lamp. The surface-protected Cu 2 O photocathode was immersed in an aqueous solution containing 0.2 mM (NH 4 ) 2 MoS 4 and 0.1 M NaClO 4 (pH 6.8). The MoS 2+ x catalyst was deposited following two routes: in the first route, consecutive cyclic voltammograms (typically 160 cycles) were carried out between 0.2 and 1.7 V versus the reversible hydrogen electrode (RHE) at a scan rate of 0.05 V s −1 starting and ending at the cathodic potential ( Supplementary Fig. 1 ). This photocathode is denoted as MoS 2+ x -CV-Cu 2 O. The second route consisted of an anodic photoelectrodeposition at a constant potential of 1.7 V versus RHE (MoS 2+ x -CA-Cu 2 O) during 150 min. Figure 1b is a photograph of this photoelectrode. It should be noted that no oxidative deposition occurs when a KG3 infrared/ultraviolet filter is interposed between the light source and the photoabsorber (inset in Supplementary Fig. 1a ). Thus, oxidation processes in the multilayer photocathode depend on the absorption of short wavelength photons (<380 nm) that generate holes in the TiO 2 overlayer ( vide infra ). Characterization of the surface-protected Cu 2 O before and after deposition of the MoS 2+ x catalyst indicates the formation of a conformal HER catalyst film ( Fig. 2 and Supplementary Fig. 2 ). The thin Cu 2 O films used for this study consist of a thin film of 400 nm finished by surface grains with an average size of 273 nm. Grain size distribution was determined by analysis of scanning electron microscopy (SEM) images before HER catalyst deposition as shown in the Supplementary Fig. 3 . The SEM cross-section image of the MoS 2+ x -CV-Cu 2 O photocathode in Fig. 2c shows a thick layer ( ∼ 50–100 nm) of MoS 2+ x deposited on top of the AZO and TiO 2 -protective layers. Wide-range XPS analysis of the photocathode surface indicates the presence of mainly Mo and S and the absence of Ti, Cu or Zn, further confirming the creation of a conformal film of at least 10 nm thick on top of the layered device ( Supplementary Fig. 4 ). The XPS spectra of the as-prepared molybdenum sulphide catalysts on Cu 2 O are similar to those earlier deposited by electrochemical methods on a FTO electrode ( Supplementary Fig. 5 ) [18] . Detailed description of XPS data fitting is given in Supplementary Note S1 and Supplementary Tables 1 and 2 . The precatalyst in MoS 2+ x -CA-Cu 2 O resembles MoS 3 , whereas that in MoS 2+ x -CV-Cu 2 O films resembles MoS 2+ x (ref. 20 ). In agreement with our previous observations for electrocatalytic hydrogen evolution [20] , the precatalyst in MoS 2+ x -CA-Cu 2 O is transformed into MoS 2+ x during photocatalysis ( vide infra ). 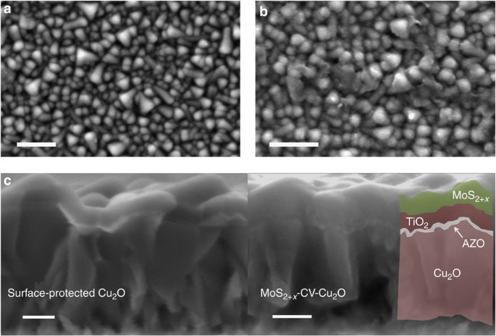Figure 2: SEM images of thin-film Cu2O photocathodes. (a) Surface-protected photocathode before HER catalyst deposition. Scale bar, 1 μm. (b) Photocathode after MoS2+xcatalyst photoelectrochemical deposition by cyclic voltammetry (CV) and activation for H2evolution for 1 h at pH 1.0. Scale bar, 1 μm. (c, left) Cross-sectional SEM image of the protective layers (20 nm AZO and 100 nm TiO2) on Cu2O and (right) aca. 100 nm of MoS2+xfilm on top of the protected Cu2O electrode. Scale bars, 200 nm. Figure 2: SEM images of thin-film Cu 2 O photocathodes. ( a ) Surface-protected photocathode before HER catalyst deposition. Scale bar, 1 μm. ( b ) Photocathode after MoS 2+ x catalyst photoelectrochemical deposition by cyclic voltammetry (CV) and activation for H 2 evolution for 1 h at pH 1.0. Scale bar, 1 μm. ( c , left) Cross-sectional SEM image of the protective layers (20 nm AZO and 100 nm TiO 2 ) on Cu 2 O and (right) a ca . 100 nm of MoS 2+ x film on top of the protected Cu 2 O electrode. Scale bars, 200 nm. Full size image PEC hydrogen evolution properties The MoS 2+ x -Cu 2 O photocathodes were tested for hydrogen evolution under simulated AM 1.5 solar illumination. Thorough characterization of the photovoltaic properties of the surface-protected Cu 2 O photocathode utilizing a RuO x catalyst, including the incident-photon-to-current efficiency and validation of the light source, has been previously reported [23] . 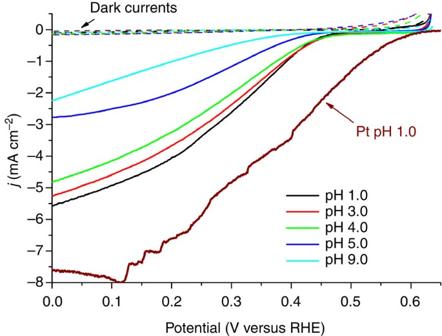Figure 3: Solar-driven PEC hydrogen evolution. Current–potential curves at different pH values for a MoS2+x-CV-Cu2O photocathode (10th scan). Scan rate is 10 mV s−1in the cathodic direction. The geometric surface area is 0.3 cm2and the catalyst loading is 30 μg cm−2. Figure 3 displays the current–potential curves in the dark and under illumination for a MoS 2+ x -CV-Cu 2 O photocathode (catalyst loading 30 μg cm −2 ). A photocurrent of −5.7 mA cm −2 at 0 V versus RHE (that is, no thermodynamic bias) was obtained at pH=1. The onset potential of photocurrent is +0.45 V versus RHE and the dark currents are negligible. Similar currents were obtained for the MoS 2+ x -CA-Cu 2 O photocathode ( Supplementary Fig. 6a ). The activity of MoS 2+ x is comparable to Pt and RuO x deposited on the same photocathode ( Supplementary Table 3 ). The early-onset potential is noteworthy and reflects the high photovoltage provided by the Cu 2 O/AZO junction. Comparison with a similar Cu 2 O photocathode loaded with Pt nanoparticles shows a difference of 150 mV for the onset potential. This is in agreement with the activity of amorphous MoS 2+ x and Pt for electrochemical hydrogen evolution [18] . [8] Seger et al. also found that the onset potential of a MoS x catalyst is 145 mV more negative than that of Pt on a Ti- n + p -Si photoelectrode [13] . Figure 3: Solar-driven PEC hydrogen evolution. Current–potential curves at different pH values for a MoS 2+ x -CV-Cu 2 O photocathode (10th scan). Scan rate is 10 mV s −1 in the cathodic direction. The geometric surface area is 0.3 cm 2 and the catalyst loading is 30 μg cm −2 . Full size image Interestingly, the MoS 2+ x catalyst is active for PEC hydrogen evolution under both acid and slightly basic conditions. From pH=1.0 to 4.0, and with the same catalyst loading of 30 μg cm −2 , only a small decrease in photocurrents was observed. Increasing pH further decreased significantly the photocurrent. Still, a substantial current density of −2.3 mA cm −2 could be obtained at pH=9.0 at 0 V versus RHE. The decrease of photocurrent and worsening of the fill factor at higher pHs is consistent with the electrochemical activity of MoS 2+ x films grown on FTO ( Supplementary Fig. 7 ) [18] . The photocurrents at high pH, however, can be increased by applying a higher loading of catalyst ( Supplementary Fig. 8 ). At pH=5.0, a photocurrent of −4.5 mA cm −2 was obtained with a MoS 2+ x loading of 50–70 μg cm −2 . At an even higher loading of catalyst, however, the photocurrent decreased, which is probably because of the absorption of light by the MoS 2+ x film that decreases the irradiation on the Cu 2 O electrode [18] . At pH=1.0 and within the range of 20–50 μg cm −2 of MoS 2+ x loading, the photocurrents are independent of catalyst loading, probably because at this pH the extraction of excited electrons by the HER catalyst is so efficient that it is already maximized at a low loading. The fast electron extraction by the MoS 2+ x film at pH 1.0 is evident, as the transient behaviour is not observed under chopped light illumination at potentials negative of 0.3 V versus RHE ( Supplementary Fig. 6b ). Similar to pH=5.0, the photocurrent decreased when the loading exceeded 50 μg cm −2 , again probably because of the absorption of light by the catalyst. The coupling of HER catalysts to semiconductor devices requires a compromise between higher surface area with higher catalyst loadings and the degree of incident light absorbed or reflected by the catalyst [3] . The contributions to the photocurrent due to photon absorption by the TiO 2 -protective overlayer and the MoS 2+ x are negligible under simulated AM 1.5 illumination. As a control experiment, the current behaviour under light and in the dark for a dummy photocathode consisting of only a MoS 2+ x film grown on 100 nm of TiO 2 was measured at 0 V versus RHE ( Supplementary Fig. 9a ). The photocurrents are three orders of magnitude smaller than the photocurrents observed under the same conditions for the MoS 2+ x -CA-Cu 2 O and MoS 2+ x -CV-Cu 2 O photocathodes. The spectrum of light reaching the photocathode shown in Supplementary Fig. 9b resembles closely the AM 1.5 G solar spectrum where the contribution of wavelengths in the near-ultraviolet region that could excite electrons over the TiO 2 band gap is small. The preparation of the photocathodes and the performance observed are reproducible and the results shown here correspond to the compilation of data obtained for more than 40 photocathodes prepared in more than seven different batches during a period of 6 months. The current densities are independent of the area covered with catalyst and exposed to illumination. The active areas of the photocathodes varied from 0.2 to 0.8 cm 2 without any noticeable difference in performance per unit area. The photocurrents measured under optimized conditions (−5.7 mA cm −2 at 0 V versus RHE and pH 1.0) are the same as previously reported with the RuO x catalyst at pH 5 (ref. 23 ). To the best of our knowledge, this value is the highest ever reported for a Cu 2 O material without the use of noble-metal HER catalysts ( Supplementary Table S4 ). Previous efforts to produce hydrogen from NiO x -coated p -Cu 2 O (ref. 16 ) and carbon-protected p -Cu 2 O (ref. 14 ) photoelectrodes have shown initial photocurrent densities of −4.98 and −3.95 mA cm −2 , respectively, at 0 V versus RHE. 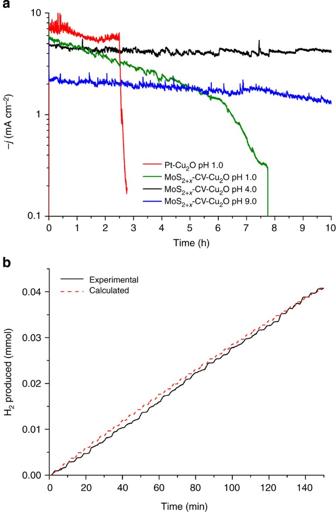Figure 4: Long-term stability and Faradaic efficiency. (a) Photocathode stability at 0 V versus RHE for Cu2O photocathodes modified by different HER catalysts under constant AM 1.5 illumination. (b) Calculated versus real hydrogen production using a MoS2+x-CA-Cu2O photocathode (biased at 0 V versus RHE) under chopped AM 1.5 irradiation at pH 4.0. The theoretical and experimental values represent the expected and observed amount of H2produced, assuming a quantitative Faradaic yield for H2formation after an activation process of 20 min. Although these photocathodes show remarkable initial photocurrent, they quickly deactivate over a period of 20 min and show low Faradaic efficiency ( Supplementary Table 4 ). Photocathode stability and Faradaic efficiency Long-term photocatalytic hydrogen evolution measurements under simulated AM 1.5 illumination show that the use of MoS 2+ x as HER catalyst increases the stability of the photocathode ( Fig. 4a ). At pH=4.0, the photocurrent is stable at −4.5 mA cm −2 for 10 h under continuous illumination for a MoS 2+ x -CV-Cu 2 O photocathode. The MoS 2+ x -CV-Cu 2 O photocathode is also stable at pH 9.0 and a substantial current density of −2.0 mA cm −2 was observed during 10 h. At pH=1.0, the photocurrent gradually decreases to below −1 mA cm −2 after 7 h. On the contrary, the photocurrents from a Pt-Cu 2 O photocathode are less stable. At pH=5.0, it was shown earlier that only 62% of the initial photocurrent was conserved after 10 h of testing under chopped light [22] ; at pH=1.0, the current erodes within 3 h according to the current study ( Fig. 4a ). Figure 4: Long-term stability and Faradaic efficiency. ( a ) Photocathode stability at 0 V versus RHE for Cu 2 O photocathodes modified by different HER catalysts under constant AM 1.5 illumination. ( b ) Calculated versus real hydrogen production using a MoS 2+ x -CA-Cu 2 O photocathode (biased at 0 V versus RHE) under chopped AM 1.5 irradiation at pH 4.0. The theoretical and experimental values represent the expected and observed amount of H 2 produced, assuming a quantitative Faradaic yield for H 2 formation after an activation process of 20 min. Full size image The decrease of the photocurrent of TiO 2 -protected Cu 2 O photocathodes is normally attributed to three main factors: (i) the dissolution of the amorphous TiO 2 by acid; (ii) the formation of Ti 3+ electron traps in the titania film; and (iii) the detachment of the HER catalyst during photoelectrolysis [8] , [10] . Whereas Pt islands do not prevent the corrosion of TiO 2 , MoS 2+ x films seem to form a conformal layer that better isolates the inner layers from the solution, reducing the contact between TiO 2 and acid. This is consistent with the cross-section SEM images of the MoS 2+ x -CV-Cu 2 O photocathode ( Fig. 2c ). Furthermore, amorphous MoS 2+ x films are stable in strongly acidic conditions [18] and SEM shows that a thin layer of MoS 2+ x remains on the surface of the photocathodes after 1 h of photolytic HER ( Supplementary Fig. 2c,g ). It should be noted that the stability issues of Pt-Cu 2 O photocathodes are not due to the lower stability of Pt catalyst but due to the detachment of Pt nanoparticles from the TiO 2 surface (pH=5.0) [22] and the dissolution of the TiO 2 layer (pH=1.0). PEC measurements of protected Cu 2 O without a HER catalyst showed that the TiO 2 layer dissolved over time at pH 1.0 while it is stable at pH 4.0 ( Supplementary Fig. 10 ). The deposition of protective layers different from TiO 2 with a higher stability in acid might further improve the stability of the whole device. Recently, [17] Laursen et al. demonstrated that MoS 2 , a more stable material than TiO 2 in acid, can act as a protective layer when grown directly on n + p -Si photocathodes [17] . Hydrogen production efficiency of a MoS 2+ x -CA-Cu 2 O photocathode under AM 1.5 illumination was probed at pH 4.0 ( Fig. 4b ). A stable photocurrent density was obtained under illumination, whereas the dark current was negligible at 0 V versus RHE ( Supplementary Fig. 11a ). Bulk photoelectrolysis shows a Faradaic efficiency close to 100% after a small induction period of 20 min ( Fig. 4b and Supplementary Fig. 11b ). The induction time is associated with the reduction of MoS 3 to the active phase of MoS 2+ x (see Supplementary Note S1 for detailed XPS characterization) and the dissolution of the initially produced H 2 in the air-saturated electrolyte. The Mott–Schottky analysis for the different layers of the device was used to determine the flat band potential and estimate the dopant density in the near-surface region (see Supplementary Note S2 and Supplementary Figs 12 and 13 ). 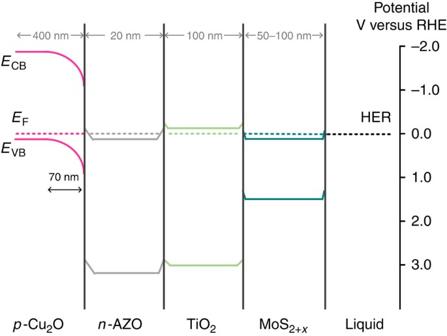Figure 5: Band energy diagram. Band energy positions for the Cu2O photocathode with Al-doped ZnO (AZO) and TiO2overlayers and the MoS2+xcatalyst film biased at 0 V versus RHE in the dark assuming pinning of the band edges of the semiconductor at the interfaces. Figure 5 shows the schematic relative band position for the multijunction photocathode after equilibration in the dark assuming band edge pinning at the interfaces and taking the built-in potentials at the interfaces equal to the difference in Fermi level [22] . The electrochemical potential of the solution is taken as the HER level, which is true under conditions of hydrogen evolution at the photocathode. The band position diagram in Fig. 5 explains many of the characteristic features observed in this device. First, the layered structure cannot drive any oxidative deposition of the HER catalyst in the semiconductor–electrolyte interface in the absence of high-energy photons. The high-potential barrier at the n -AZO and the p -Cu 2 O interface prevents any electrons from flowing from the TiO 2 to the Cu 2 O layer through the valence band. The absorption of high-energy photons by the TiO 2 from the unfiltered Xe lamp creates holes that drive oxidative PEC deposition of the MoS 2+ x catalyst. Photoexcited electrons avoid recombination and flow through the conduction band of the overlayers into the Cu 2 O valence band when the photocathode is biased at potentials more positive than the flat band potential of the Cu 2 O layer (+0.81 V versus RHE, Supplementary Table 5 ) as observed in the inset of Supplementary Fig. 1a and depicted in Supplementary Fig. S14 . Second, the conduction band of the n -type AZO, TiO 2 and MoS 2+ x have a position more reductive than the HER potential, which is favourable for the conduction of photogenerated electrons in the photocathode as confirmed by this work ( Supplementary Fig. 14a ). The photovoltage of the buried p–n junction has been experimentally found to be between 0.5 and 0.6 V (ref. 23 ). This explains the onset potential for hydrogen evolution at +0.6 V observed for Pt on this photocathode and +0.45 V for the MoS 2+ x catalyst. Figure 5: Band energy diagram. Band energy positions for the Cu 2 O photocathode with Al-doped ZnO (AZO) and TiO 2 overlayers and the MoS 2+ x catalyst film biased at 0 V versus RHE in the dark assuming pinning of the band edges of the semiconductor at the interfaces. Full size image In summary, we have successfully deposited MoS 2+ x films as a HER catalyst on TiO 2 -protected Cu 2 O photocathodes. The catalyst displays many features that are desirable for a PEC water-splitting device: simple and scalable process of deposition, optical transparency, stability during 10 h of continuous operation and low overpotential for the HER. The integrated device produces photocurrents as high as −5.7 mA cm −2 at 0 V versus RHE (photocurrents that would correspond to 7% STH efficiency in a tandem cell configuration) with a ∼ 100% Faradaic yield. Moreover, the layered device reported here is the most active Cu 2 O photocathode to date that makes use of an earth-abundant HER catalyst ( Supplementary Tables 3 and 4 ). General considerations All manipulations were carried out under atmospheric conditions, unless otherwise mentioned. All reagents were purchased from commercial sources and used without further purification. Millipore deionized water 18.2 MΩ was used to prepare all the solutions. Cu 2 O electrodeposition The Cu 2 O thin films were deposited by electrodeposition from a basic solution of lactate-stabilized copper sulphate as previously reported by one of our groups [10] . In brief, Cu 2 O thin films were deposited in a plating bath kept at 30 °C using a potentiostat (IviumStat) in a two-electrode configuration cell at a constant current density of −0.1 mA cm −2 (galvanostatic mode) for 105 min. The deposition electrode was a 70 × 30 mm 2 TEC-15 fluorine-doped tin oxide (FTO; Nippon Sheet Glass) coated with 10 nm Cr and 150 nm of Au (deposited by sputtering) and the counter electrode was a 25 × 25 mm 2 Ti metal plate. The titanium counter electrode was used to avoid any Pt contamination of the device. The plating bath was an aqueous 0.2 M CuSO 4 (Sigma-Aldrich, 98+%) and 3 M lactic acid (Roth, 90%) solution with 0.5 M K 2 HPO 4 (Sigma, 98+%) buffer. The bath pH was adjusted to pH 12 using a 2 M KOH (Reactolab) solution. The plating bath concentrations refer to the initial bath concentration before pH adjustment. Atomic layer deposition ALD was used to deposit ultrathin layers of n -type oxides on the surface of the Cu 2 O thin films using a thermal ALD system (Savannah 100, Cambridge Nanotech). The general conditions for ALD have been optimized and reported by Paracchino et al. [22] Typically, the ALD of Al:ZnO (AZO) was carried out at a substrate temperature of 120 °C. The precursors were diethyl zinc (ABCR, 95%), trimethyl aluminium (ABCR, 98%) and H 2 O kept at room temperature as the Zn, Al and O precursors, respectively. Each precursor was held in the chamber for 2.0 s, followed by a 15-s nitrogen purge. Aluminium-doped ZnO (Al:ZnO) was deposited by intercalating one cycle of trimethyl aluminium and water after 20 cycles of diethyl zinc and water. The growth rate per cycle under these conditions was previously determined to be 1.7 and 2.0 Å for Al 2 O 3 and ZnO, respectively. TiO 2 was deposited at a substrate temperature of 150 °C using tetrakis-(dimethylamino)titanium (99.99%, Aldrich), at a precursor temperature of 75 °C, and hydrogen peroxide (50% in water, stabilized, Aldrich) at room temperature. TiO 2 was deposited in pulse mode under a nitrogen flow of 5 s.c.c.m., with a pulse length of 0.1 s and wait period of 10 s for both precursors. The growth rate per cycle for TiO 2 was determined by ellipsometry on a silicon wafer with native oxide and corresponded to 0.58 Å per cycle at 150 °C. MoS 2+ x HER catalyst PEC deposition The deposition of MoS 2+ x catalyst on the Cu 2 O photocathode coated with AZO and TiO 2 overlayers was done under non-filtered irradiation from a 180-W Xe lamp (Osram). The illumination intensity on the deposition cell was 130 mW cm −2 . Epoxy resin or Teflon tape was used to cover any Au or FTO substrate exposed and to limit the area of catalyst deposition. A freshly prepared photocathode was immersed into a 0.2-mM aqueous solution of (NH 4 ) 2 MoS 4 (Aldrich, 99.97%) in 0.1 M NaClO 4 (ABCR, 99%) at a pH of 6.8. Both chemicals were used as received. The MoS 2+ x catalyst was deposited following two routes: in the first route, consecutive cyclic voltammograms (typically 160) were carried out on an IviumStat potentiostat (Ivium Technologies) with a saturated Ag/AgCl reference electrode (separated by a porous silica gel frit) and a Ti wire counter electrode. The cyclic voltammograms were performed between 0.2 and 1.7 V versus RHE at a scan rate of 0.05 V s −1 starting and ending at the cathodic potential (photocathode identified as MoS 2+ x -CV-Cu 2 O). The second method consisted of the same conditions as described above, but instead of consecutive voltammograms, a constant potential of 1.7 V versus RHE was applied for different periods of time (photocathode identified as MoS 2+ x -CA-Cu 2 O). For the Mott–Schottky analysis and study of the contribution to the photocurrent from photon absorption by the TiO 2 , the same procedure was used to deposit MoS 2+ x catalyst films on electrodes consisting of a 100-nm TiO 2 layer grown by ALD on FTO. Pt nanoparticles deposition on surface-protected Cu 2 O Platinum nanoparticles were galvanostatically electrodeposited in the dark from a 1 mM aqueous solution of H 2 PtCl 6 (ABCR, 99.9%; pH=2.4). A current density of −8.5 μA cm −2 was kept during 15 min (ref. 22 ). Physical and chemical characterization The electrodes were characterized by SEM and XPS. SEM secondary electron images were taken on a Philips (FEI) XLF-30 field emission gun SEM. ImageJ software was used to measure the distances in SEM images. XPS data were collected on an Axis Ultra instrument (Kratos Analytical) under ultrahigh vacuum (<10 −8 torr) using a monochromatic Al K α X-ray source (1,486.6 eV), in the Surface Analysis Laboratory of Interdisciplinary Center for Electron Microscopy at Ecole Polytechnique Fédéerale de Lausanne. The source power was maintained at 150 W (10 mA, 15 kV). The adventitious carbon 1 s peak was calibrated at 284.8 eV and used as an internal standard to compensate for any charging effects. Both curve fitting of the spectra and quantification were carried out with the CasaXPS software using relative sensitivity factors from the supplier. PEC measurements PEC measurements were recorded by an IviumStat electrochemical analyser. A three-electrode configuration under front-side simulated AM 1.5 illumination was used where a Pt wire was used as the counter electrode and an Ag/AgCl (KCl sat.) electrode was used as the reference electrode. Different electrolyte buffer solutions were used at different pH values and were referenced in the text by the pH value unless otherwise mentioned. pH 5.0 solution consisted of a 1.0 M Na 2 SO 4 (Sial, 99+%) buffered with 0.1 M K 3 PO 4 (Aldrich, 97%). pH 4.0 solution consisted of 0.5 M Na 2 SO 4 with 0.2 M potassium hydrogen phthalate (Fluka, 99.5+%) buffer. Solutions of 0.5 M Na 2 SO 4 buffered with 0.1 M formic acid (Merck, 98–100%) and 0.1 M phosphoric acid (ABCR, 98%) were used as pH 3.0 and 2.0 buffer solution, respectively. pH 9.0 solution consisted of 0.1 M sodium tetraborate (Sial, 99.5+%). Finally, 0.1 M H 2 SO 4 (Merck, 95–97%) was used as pH 1.0 and 0.1 M NaOH (Riedel, 98–100%) was used as pH 12.9 solutions. The photoresponse was measured under irradiation from a 450-W Xe lamp (Osram) equipped with a KG3 filter (3 mm, Schott, filters ultraviolet and infrared light; see Supplementary Fig. S9b ), calibrated with a Si diode to simulate AM 1.5 illumination (100 mW cm −2 =1 sun). The scan rate for the linear sweep voltammetry was 10 mV s −1 in the cathodic direction. Photocurrent stability test were carried out by measuring the photocurrent produced under constant light irradiation at a fixed electrode potential of 0 V versus RHE. During linear sweep voltammetry ( j –V plots) and chronoamperometry (stability plots), the electrolyte was continuously bubbled with N 2 to remove oxygen and thus eliminate erroneous signals arising from oxygen reduction. The electrochemical impedance spectroscopy (EIS) measurements were carried out using an Autolab potentiostat/galvanostat. Impedance measurements on freshly electrodeposited Cu 2 O films were carried out in the dark using a three-electrode configuration. The electrolyte was 0.1 M sodium acetate (Aldrich, 99+%; pH 7.85) in water. The potential was swept in the range of stability predicted by the Pourbaix diagram (0.4–0.6 V versus RHE) and an alternate current signal of 10 mV of amplitude was superposed on the direct current component. Before EIS measurements, the electrode was dipped for 15 s in a 0.8 M acetic acid solution to remove the native CuO layer on the surface. EIS measurements for ALD TiO 2 (100 nm) on FTO were carried out in a 0.1 M NaOH (pH 12.9) between 0.5 and 1.0 V versus RHE. Impedance measurements for MoS 2+ x on TiO 2 (100 nm) were carried out in the KHP buffer solution (pH 4.0). EIS experimental data were analysed and fitted using ZView software (Scribner Associates). Hydrogen measurements were taken in a manner similar to the photocurrent measurements at a constant potential of 0 V versus RHE under chopped 1 sun AM 1.5 illumination in a H cell calibrated for hydrogen evolution measurements as described in the literature and adapted with a optically transparent window for light irradiation [25] . The electrolyte used was KHP buffer solution (pH 4.0). The Faradaic efficiency was calculated from the total amount of charge Q (C) passed through the cell and the total amount of hydrogen produced n H2 (mol). The total charge was obtained from the integration of the measured current. The total amount of hydrogen produced was measured using a calibrated pressure sensor. For the reduction of protons, two electrons are needed to reduce two protons and produce one H 2 molecule. Thus, the Faradaic efficiency can be calculated using the equation, Faradaic efficiency= n H2 /( Q /2 F ), where F is the Faraday constant. Stability tests were carried out in a manner similar to the photocurrent measurements at a constant potential of 0 V versus RHE with constant nitrogen overflow. Light source spectra determination Light source spectra were obtained using an Ocean Optics USB2000+ Fiber Optic Spectrometer (responsive from 200 to 1,100 nm) with SpectraSuite software. The irradiance of the light source with and without the KG3 filtre was measured using the irradiance of an Osram HLX 64623 halogen bulb (colour temperature=3,200 K) as a standard. How to cite this article: Morales-Guio, C. G. et al. Hydrogen evolution from a copper(I) oxide photocathode coated with an amorphous molybdenum sulphide catalyst. Nat. Commun. 5:3059 doi: 10.1038/ncomms4059 (2014).